Humans and chimpanzees attend differently to goal-directed actions Humans comprehend the actions of others by making inferences about intentional mental states of another. However, little is known about how this capacity develops and whether this is shared with other animals. Here we show the ontogenetic and evolutionary foundations of this ability by comparing the eye movements of 8- and 12-month-old human infants, adults and chimpanzees as they watched videos presenting goal-directed and non-goal-directed actions by an actor. We find that chimpanzees anticipate action goals in the same way as do human adults. Humans and chimpanzees, however, scan goal-directed actions differently. Humans, particularly infants, refer to actors' faces significantly more than do chimpanzees. In human adults, attentional allocation to an actor's face changes as the goal-directed actions proceed. In the case of non-goal-directed actions, human adults attend less often to faces relative to goal-directed actions. These findings indicate that humans have a predisposition to observe goal-directed actions by integrating information from the actor. Humans have a strong tendency to view the actions of others not simply as physical movements, but rather as reflecting intentional mental states, for example, beliefs about the world, desires for things. One of the ways to attribute intentional mental states to others from observing their action involves interpreting the action as goal-directed. Understanding actions as goal-directed is crucial for predicting the effects or outcome of the actions. We make inferences about the action goals of an individual by assessing the end state that would be efficiently brought about by their actions, given particular situational constraints [1] , [2] , [3] . If we observe an actor, holding books in both hands and turning on a light switch with his forehead, we interpret this action as goal-directed, given constraints on using his hands. However, if the same forehead-switch action occurs while both hands are free, it strikes us as less purposeful [4] . Ontogenetically, this capacity emerges as early as 6.5 months of age [5] . Recent studies have revealed the evolutionary roots of this capacity in other primates. Chimpanzees ( Pan troglodytes ) [6] and macaque monkeys ( Macaca nemestrina, M. fascicularis and M. mulatta ) [7] also possess the ability to evaluate the efficacy of other individuals' goal-related actions. How do humans and other primates evaluate the adequacy of goal-directed actions? One possible explanation is that other individuals' actions are understood through a direct matching process of a mirror neuron system, where an observed action is mapped onto the observers' own motor representation of that action [8] , [9] , [10] . According to the direct-matching hypothesis, the prediction of another's action goals is closely related to the observer's own action repertoire. Recent developmental studies support this view by suggesting that the onset age of infants' ability to predict goal-directedness is synchronized with the onset age of their own ability to perform that action [11] , [12] . At around 6 months of age, for example, human infants interpret grasping responses, which are actions within those possible at this age, as goal-directed [13] . Other cues for understanding actions derive from attentional or emotional information, such as the direction of gaze and facial expressions of other individuals. Such referential information directs an observer's attention to specific objects or to specific aspects of the environment on the basis of understanding particular relations that link these referential cues to their referents. Previous studies have shown that by 12–14 months of age, infants begin to use information about others' gaze direction and emotional expression to predict an action goal [14] , [15] , [16] . For example, a human infant watches an actress looking with gaze direction and emotional expressions at an object A, and then, is subsequently shown this actress holding the same object A or a different object B. Typically, an infant will look longer at the event where the actress holds the object B than the event where the actress holds the object A [14] . This result can be interpreted as suggesting that infants use referential information to predict the action goal of another individual. Several studies have reported that non-human primates also use referential information [17] , [18] , [19] , [20] , [21] . When young nursery-reared chimpanzees are exposed to a novel object, they exhibit gaze alternation between this object and the face of their primary caregiver, a phenomenon similar to human social referencing [17] . Recent eye-tracking studies have illustrated that chimpanzees and macaques are attracted to the face and eye regions of both human and non-human animals [22] , [23] . Chimpanzees look at the face region longer than at other parts of a body when they are presented with various still photographs depicting human and non-human animals, although the degree to which they look at the faces is somewhat lower than in the case of human adults [22] . However, these findings on social referencing and saliency of the face region do not explain how non-human primates might use referential information for understanding others' actions. We have little knowledge about how humans and non-human primates look at sequential, dynamic actions of other individuals. Previous studies on human infants, for example, have mainly used habituation/dishabituation or preferential looking paradigms; however, these methodologies are limited in their potential for revealing an extent to which infants actually track the observed actions or faces of others. An eye-tracking technique enables us to investigate this issue by assessing eye movements as a sequence of observed actions unfolds. Exploring the extent to which humans and non-human primates are similar and different in their respective viewing of others' actions can contribute to discovering the evolutionary foundation of the human ability for intentional understanding of others' actions. The current series of experiments uses eye-tracking technology, which has been rarely applied to non-human primates. One aim was to investigate the styles of attending to others' goal-directed actions in humans and chimpanzees, humans' closest living relatives. A second aim, which addresses issues of the human ontogeny of action understanding, involved a comparison of the eye movements of 8- and 12-month-old human infants and adults. We investigated developmental changes in the visual patterns of the eye movements associated with a goal-directed action, as these relate to a hypothesized age-specific capacity to perform the same action themselves. According to the direct-matching hypothesis, visual scanning patterns for an action should depend upon the motor ability of the observer to perform this action. Also, if attentional referential information such as other's gaze direction is processed along with the process of encoding goal-directedness of an action, then the behaviour of looking at the faces, which can be quantified by the eye-tracking, should change as the goal-directed action proceeds. We show that chimpanzees anticipate action goals in the same way as human adults. However, chimpanzees and humans, particularly human infants, differ in how they direct attention to others' goal-directed actions. Visual scanning patterns for a goal-directed action In Experiment 1, we investigated the gaze behaviour of human adults ( n =15), 8-month-old human infants ( n =15), 12-month-old human infants ( n =14) and chimpanzees ( n =6) during video presentations showing two identical trials, in which a human demonstrator (actor) performed the goal-directed action of pouring juice into a cup. Adults and chimpanzees can produce this action by themselves. The 12-month-old, but not the 8-month-old, infants can perform similar, but simpler, versions of this action (that is, placing one object in a container into another container). An eye tracker was used to assess whether participants expected (shown by anticipatory eye movements) the action goal before the goal was achieved [11] (latency to fixate on the cup relative to the onset of pouring), and whether participants referred to the actor's face (ratio of looking time, number of fixations and fixation duration among the four areas of interest (AOIs) combined (cup, trajectory (moving juice bottle), face and other)) while viewing the action ( Fig. 1a , Supplementary Movie 1 ). 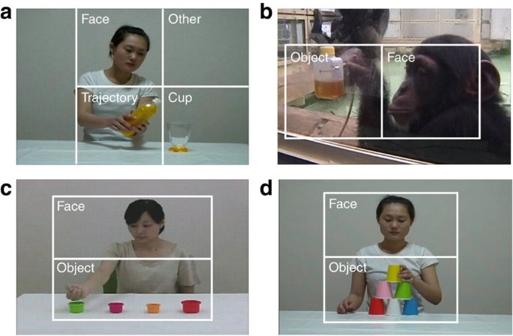Figure 1: A selected scene from the video stimulus used in each experiment and areas of interest for analysis. (a) Experiment 1: an adult female human actor, sitting in front of a table, pouring some juice from a bottle into a clear glass cup. The video lasted 14.0 s. (b) Experiment 2: a captive chimpanzee (male) inserting a rubber tube into a small hole in a transparent wall to fish for honey in a container attached to the opposite side of the wall. The chimpanzee actor was unfamiliar to human and chimpanzee participants. The video lasted 8.0 s. (c) Experiment 3: an adult female human sitting at a table and reaching towards, but not grasping, four cups with the palm facing upwards in a manner that appeared, from a human perspective, non-goal-directed. The video lasted 15.0 s. (d) Experiment 4: an adult female sitting at a table and stacking six cups. The video lasted 13.0 s. Figure 1: A selected scene from the video stimulus used in each experiment and areas of interest for analysis. ( a ) Experiment 1: an adult female human actor, sitting in front of a table, pouring some juice from a bottle into a clear glass cup. The video lasted 14.0 s. ( b ) Experiment 2: a captive chimpanzee (male) inserting a rubber tube into a small hole in a transparent wall to fish for honey in a container attached to the opposite side of the wall. The chimpanzee actor was unfamiliar to human and chimpanzee participants. The video lasted 8.0 s. ( c ) Experiment 3: an adult female human sitting at a table and reaching towards, but not grasping, four cups with the palm facing upwards in a manner that appeared, from a human perspective, non-goal-directed. The video lasted 15.0 s. ( d ) Experiment 4: an adult female sitting at a table and stacking six cups. The video lasted 13.0 s. Full size image Predictive eye movements Latency data were tested against 0 ms (defined as the onset of pouring juice) to assess whether performance was significantly predictive (positive latencies, ms) or reactive (negative latencies, ms). Adults (mean=787.37, t 14 =4.71, P =0.001, Cohen's d =1.72) and chimpanzees (mean=843.33, t 5 =5.71, P =0.002, Cohen's d =3.29), on average, shifted their gaze to the goal before the juice was poured into the cup, whereas 12-month-olds did not (mean=61.25, t 13 =0.20, P =0.84). Eight-month-olds did so after the juice was poured into the cup (mean=−2,606.41, t 10 =−3.90, P =0.003, Cohen's d =−1.66; Fig. 2 ). Comparison across the four groups revealed a significant effect on predictive eye movements to the goal (F 3,45 =16.60, P <0.001, η 2 =0.30). Post-hoc testing (Bonferroni) showed that 8-month-olds differed from the other three groups ( P s<0.001 in all cases), whereas differences among the latter three groups were not significant. 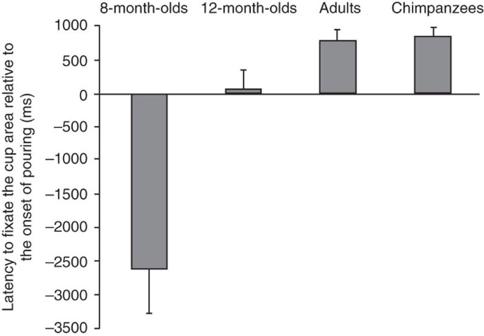Figure 2: Latency to fixate on the goal relative to defined zero point. Latency to fixate on the cup area (goal) relative to the onset of pouring juice into the cup (defined as a zero point). Positive values correspond to fixation shifts to the cup before the onset of pouring. Error bars represent s.e.m. Figure 2: Latency to fixate on the goal relative to defined zero point. Latency to fixate on the cup area (goal) relative to the onset of pouring juice into the cup (defined as a zero point). Positive values correspond to fixation shifts to the cup before the onset of pouring. Error bars represent s.e.m. Full size image Spatial distribution and duration of fixations The spatial distribution of fixations revealed a visual scanning pattern, which differed from that found in predictive eye movements. A 2 (phase: before goal, after goal)×4 (area: face, cup, trajectory, other)×4 (group: 8-, 12-month-olds, adults, chimpanzees) mixed factorial analysis of variance (ANOVA) revealed a significant three-way interaction of phase, area and group (F 9,138 =3.88, P <0.001, η 2 =0.20). The follow-up 4 (area)×4 (group) mixed ANOVA for the before-goal phase revealed a significant interaction between the area and group (F 9,138 =9.83, P <0.001, η 2 =0.39). During the before-goal phase, ratios of looking time towards the face and cup areas to total looking time towards the four areas combined differed among groups (face, F 3,46 =7.25, P <0.001, η 2 =0.32; cup, F 3,46 =34.43, P <0.001, η 2 =0.69). Post-hoc testing (Bonferroni) revealed no significant difference among the three human groups in looking towards the face area, whereas these groups differed from chimpanzees, whose ratio of looking time towards the face area was significantly lower ( P s<0.01 in all cases). Conversely, the ratio of looking towards the cup area was significantly higher in chimpanzees than in all three human groups ( P s<0.01 in all cases). Among humans, this ratio was lower in 8-month-olds than in both 12-month-olds ( P <0.05) and adults ( P <0.01), and higher in adults than in 12-month-olds ( P <0.01). The follow-up 4 (area)×4 (group) mixed ANOVA for the after-goal phase revealed a significant interaction between the area and group (F 9,138 =14.62, P <0.001; η 2 =0.49). Also during the after-goal phase, the ratios of looking time towards the face and cup areas to total looking time towards the four areas combined were different among groups (face, F 3,46 =21.85, P <0.001, η 2 =0.59; cup, F 3,46 =22.24, P <0.001, η 2 =0.59). Post-hoc testing (Bonferroni) showed that the ratio of looking time towards the face area in chimpanzees was lower than in both 8-month-olds and 12-month-olds ( P s<0.001 in both cases), whereas chimpanzees were not lower in looking at the face than human adults. The ratios of looking time towards the cup area were significantly higher in both chimpanzees and adults compared with infants ( P s<0.01 in all cases; Fig. 3a ). 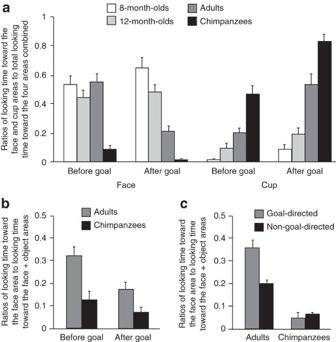Figure 3: Comparison of ratios of looking time. (a) Ratios of looking time towards the face and cup areas to total time looking towards the four areas combined before and after goal achievement in Experiment 1. (b) Ratios of looking time towards the face area to total looking time towards the combined face and object areas before and after goal achievement in Experiment 2. (c) Ratios of looking time towards the face area to total looking time towards the combined face and object areas in Experiment 1 (goal-directed action) and 3 (non-goal-directed action). Error bars represent s.e.m. Figure 3: Comparison of ratios of looking time. ( a ) Ratios of looking time towards the face and cup areas to total time looking towards the four areas combined before and after goal achievement in Experiment 1. ( b ) Ratios of looking time towards the face area to total looking time towards the combined face and object areas before and after goal achievement in Experiment 2. ( c ) Ratios of looking time towards the face area to total looking time towards the combined face and object areas in Experiment 1 (goal-directed action) and 3 (non-goal-directed action). Error bars represent s.e.m. Full size image Second, we analysed the number of fixations, which yielded findings similar to those of the ratios of looking time. A 4 (area)×4 (group) mixed ANOVA revealed a significant interaction between area and group (F 9,138 =9.51, P <0.001, η 2 =0.38). Significant group differences were found in the face and cup areas, respectively (face, F 3,46 =7.51, P <0.001, η 2 =0.33; cup, F 3.46 =25.44, P <0.001, η 2 =0.62). Chimpanzees made fewer fixations on the face area than did human infants ( P s<0.01) and adults ( P <0.05), whereas chimpanzees and adults made more fixations on the cup area than did the infants ( P s<0.01 in all cases). The third analysis of the average duration of fixations revealed further differences among groups. In general, average fixation duration for the four areas combined was shorter in chimpanzees than in human infants and adults (489 ms in chimpanzees, 597 ms in 8-month-olds, 510 ms in 12-month-olds, 615 ms in human adults), although the group main effect was not significant (F 3,46 =1.39, P =0.26). When fixations on face and object (cup and trajectory) areas were considered, a 2 (area)×4 (group) mixed ANOVA revealed a significant interaction between area and group (F 3,45 =5.52, P =0.003, η 2 =0.27). Average fixation duration on the face area differed among groups (F 3,45 =4.74, P =0.006, η 2 =0.24), being shorter in chimpanzees than in human infants and adults ( P s<0.02 in all cases); however, duration of fixations on the object area did not differ between chimpanzees and humans ( P s>0.05 in all cases). Viewing patterns for a chimpanzee's action One possible explanation for these species differences is that, for chimpanzees, the actor belonged to a different species [24] . To address this, in Experiment 2, we used a video showing a goal-directed action by a chimpanzee. The gaze behaviour of human adults ( n =13) and chimpanzees ( n =6) was investigated during two identical presentations showing a chimpanzee inserting a rubber tube into a small hole in a honey container. First, we investigated the spatial distribution of fixations on the actor's face area in relation to total time looking towards the combined face and moving object areas ( Fig. 1b , Supplementary Movie 2 ). The 2 (phase: before goal, after goal)×2 (area: face, object)×2 (group: adults, chimpanzees) mixed factorial ANOVA revealed significant two-way interactions between the phase and group (F 1,17 =8.54, P <0.01, η 2 =0.33) and between area and phase (F 1,17 =6.80, P <0.02, η 2 =0.29), but no three-way interaction (F 1,17 =1.01, P =0.33). Follow-up two-way ANOVAs were conducted separately for each phase. In the before-goal phase, the ratio of looking time towards the face area was lower in chimpanzees than in humans (F 1,17 =9.83, P =0.006, η 2 =0.37). In contrast, after the goal was achieved, the ratio of time looking towards the face area did not differ between the two groups (F 1,17 =2.62, P =0.12; Fig. 3b ). Thus, compared with chimpanzee observers, human adults paid significantly more attention to the face of a chimpanzee actor before completion of an action goal than did the chimpanzees. Second, we analysed the number of fixations, which yielded findings similar to those of the ratio of looking time. A 2 (area)×2 (group) mixed ANOVA revealed a significant interaction between the area and group (F 1,17 =30.55, P <0.001, η 2 ==0.64). The number of fixations to the face area was larger in human adults than in chimpanzees (F 1,17 =13.05, P =0.002, η 2 =0.44), whereas those to the object area was larger in chimpanzees than in humans (F 1, 17 =28.18, P <0.001, η 2 =0.62). The third analysis concerns about fixation durations. Average fixation duration for the two areas combined was shorter in chimpanzees than in humans (318 ms in chimpanzees, 446 ms in human adults; F 1,17 =17.90, P =0.001, η 2 =0.51). A 2 (area)×2 (group) mixed ANOVA revealed a significant interaction between the area and group (F 1,17 =13.06, P =0.02, η 2 =0.44). Average fixation duration on the object area was longer in humans than in chimpanzees (F 1,17 =19.99, P <0.001, η 2 =0.54). Goal-directed versus non-goal-directed actions To test the hypothesis that humans' tendency to pay attention to the face might be related to making inferences about other individuals' intentions or action goals, in Experiment 3, we investigated viewing patterns for a non-goal-directed action. The gaze behaviour of human adults ( n =15) and chimpanzees ( n =6) was investigated during a video presentation showing a human sitting at a table and reaching towards, but not grasping, four cups with the palm facing upwards, in four repetitions. We analysed the spatial distribution of fixations on the actor's face area in relation to total time looking towards the combined face and object areas ( Fig. 1c , Supplementary Movie 3 ). A 2 (area: face, object)×2 (group: adults, chimpanzees) mixed factorial ANOVA revealed a significant interaction (F 1,19 =4.85, P <0.05, η 2 =0.20). The ratio of looking time at the face area was lower in chimpanzees than in humans (F 1,19 =13.39, P =0.002, η 2 =0.41). The spatial distribution of fixations on the face areas of human actors in relation to total time looking towards the combined face and object areas for non-goal-directed action in Experiment 3 was compared with that in the goal-directed action of Experiment 1. Human adults paid more attention to the face area during presentation of a goal-directed action than a non-goal-directed action ( t 28 =3.832, P =0.001, d =1.40), whereas no such difference emerged for chimpanzees ( t 5 =−1.07, P =0.33; Fig. 3c ). 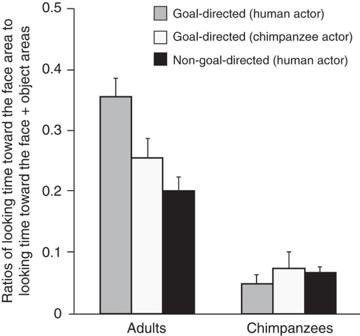Figure 4: Ratios of looking time towards the face area to total looking time towards the combined face and object areas. Goal-directed (human actor): goal-directed action by a human (Experiment 1), goal-directed (chimpanzee actor): goal-directed action by a chimpanzee (Experiment 2), non-goal-directed (human actor): non-goal-directed action by a human (Experiment 3). Note that it is not appropriate in a strict sense to compare the data across all three conditions, as the stimuli used in the three experiments were different. We used data from adults in the case of human participants, because human infants did not participate in the Experiments 2 and 3. The ratio of looking time to the face area by chimpanzees was fairly constant across the three experiments. Error bars represent s.e.m. Figure 4 additionally illustrates the result of comparison across Experiment 1, 2 and 3. Figure 4: Ratios of looking time towards the face area to total looking time towards the combined face and object areas. Goal-directed (human actor): goal-directed action by a human (Experiment 1), goal-directed (chimpanzee actor): goal-directed action by a chimpanzee (Experiment 2), non-goal-directed (human actor): non-goal-directed action by a human (Experiment 3). Note that it is not appropriate in a strict sense to compare the data across all three conditions, as the stimuli used in the three experiments were different. We used data from adults in the case of human participants, because human infants did not participate in the Experiments 2 and 3. The ratio of looking time to the face area by chimpanzees was fairly constant across the three experiments. Error bars represent s.e.m. Full size image Viewing patterns for a non-food-related action In Experiments 1 and 2, we used sequential goal-directed actions related to food as the test stimuli. We chose these actions for two reasons. First, these stimuli are quite familiar in the everyday experiences of both humans and chimpanzees serving this study [25] . Second, most object-related actions observed in wild chimpanzees (tool-using behaviours) are aimed at obtaining food [26] . However, there remains a possibility that the results of the current experiments might be because of the chimpanzees simply paying special attention to the food in the videos. To eliminate this possibility, we conducted another experiment (Experiment 4). Chimpanzees and human adults were shown another video of an adult female human sitting at a table and stacking cups; thus, this video contained no food ( Fig. 1d , Supplementary Movie 4 ). The spatial distribution of fixations differed between groups: the ratio of looking time towards the face areas was lower for chimpanzees than for humans (F 1,17 =9.59, P <0.01, η 2 =0.14). Thus, we confirmed that chimpanzees look longer at moving objects and less at the actor's face while observing object-related actions than human adults do, even when the actions are not food-related. This study obtained comparative eye-tracking data from the observers' visual scanning of dynamic object-related actions of other individuals, using both chimpanzees and humans as observers. We found that when observing actions, chimpanzees anticipate an action goal in the same way as do human adults. On the other hand, 8-month-old infants showed no evidence of goal anticipation. Twelve-month-old infants showed mixed evidence in that strong goal anticipation was not evident, but these infants did show weak predictive tendencies that were statistically comparable to those of human adults and chimpanzees. This indicates that 12-month-old infants are not yet anticipating goal-directedness as fully as human adults and chimpanzees do. According to the direct matching hypothesis [8] , [9] , [10] , these results appear to be plausible. Adults and chimpanzees can perform this action by themselves. Twelve-month-old infants, but not 8-month-old infants, can perform similar, albeit simpler, versions of this action such as placing an object in a container into another container. The results are also consistent with previous developmental studies showing that human adults and infants who are able to grasp and move an object to a container shift their gaze to the goal of the action before the hand arrives (anticipatory eye movements), whereas younger infants unable to perform the action do not shift their gaze [11] , [12] . The current findings also demonstrate that, unlike anticipatory looking patterns, visual scanning patterns of observed actions differ for chimpanzees and humans; consistent differences emerged in ratios of looking time, number of fixations and duration of fixations. In general, humans pay attention to other individuals' faces longer (ratio of looking time and fixation duration) and more frequently (number of fixations) than do chimpanzees across all situations, irrespective of goal-directed or non-goal-directed actions. Previous eye-tracking studies have found that chimpanzees pay less attention, although significantly higher than random scanning of a whole picture, to photographed faces, and that chimpanzees move their eyes more rapidly than human adults [22] , [27] . The present results offer new species differences; first, the degree of species difference gauged by the proportion of fixation to faces is larger in our study than the previous study in which participants looked at still photographs containing the whole body of human and non-human animals, although strict comparison is not possible because of methodological differences [22] . But species differences in viewing faces may be more apparent in tasks using dynamic object-directed actions of others than in tasks that require observers to merely look at still images. Second, although our data on species difference in the grand average of fixation durations are comparable to those of a previous studies (200–300 ms in chimpanzees and 200–700 ms in human adults) [22] , [27] , our results showed that the fixation durations of chimpanzees differ according to the target of fixations. When fixations to faces were considered, the average fixation duration was shorter in chimpanzees than in humans (for example, 229 ms in chimpanzees and 672 ms in human adults in Experiment 1), but the duration of fixation to the object did not differ between chimpanzees and humans (for example, 490 ms in chimpanzees and 579 ms in human adults in Experiment 1). Such results contradict with the view that chimpanzees generally move their eyes more rapidly than humans [22] , [27] ; instead, they suggest that chimpanzees change fixation durations according to contexts and that they particularly attend to the objects when they view object-directed actions of other individuals. Our most important finding is that humans' face-scanning patterns differ, depending on whether the target actions are goal-related or not. Human adults pay more attention to an actor's face while they observe a goal-direction action (versus a non-goal action), whereas chimpanzees show no difference in face-scanning patterns as a function of the two types of actions. More noteworthy is that the face-scanning patterns in human adults change as the goal-directed actions proceed. Our data indicate that after goal achievement, adults look less at the actor's face; that is, their allocation of attention to faces is greater before than after the action goal is achieved. In fact, the latter attention level is similar to that of chimpanzees. Human infants, on the other hand, continue to pay attention to the face after the action goal is achieved. These different scanning patterns cannot be attributed to the species-specific differences in general visual scanning patterns or to differential interest in faces, irrespective of goal-directedness of the observed actions [22] , [27] . Why do humans view faces especially before the goal is achieved? Why do infants continue to pay attention to the face after the goal is achieved, whereas adults do not? Our data does not provide direct answers to these questions. However, these data do suggest that attention to faces, which potentially conveys referential information such as gaze direction or emotional expression towards target object, is involved in the coding process of goal-directed actions in the case of humans. Therefore, the coding process of goal-directedness may facilitate humans' attention to the face of an actor. Humans infer goals of other individuals' actions by scanning faces while predicting the action goals. After confirming the goals, human adults may reduce their attention to the face. Infants who are still developing the ability to infer the likely goals of observed actions in everyday life, especially actions that they cannot yet perform themselves, may seek additional referential information by continuing to pay attention to the actor's face throughout. To verify these assumptions, further research is needed to confirm how and when humans' face-scanning patterns change, depending on the sequential progressing of goal-directed actions in development. In conclusion, our findings establish a quantitative difference in how humans and chimpanzees look at the goal-directed actions of others. Chimpanzees anticipate action goals in the same way as human adults do. However, these two groups differ significantly in areas to which they attend. Humans, particularly infants, attend to the actors' faces more than do chimpanzees. We assume that chimpanzees predict the action goal, depending mainly on object-related information. On the other hand, humans have a strong predisposition to view goal-directed actions by integrating information of a distinctive directedness to specific objects and the actor's referential information. Further studies are also needed to investigate developmental trajectory of visual attentional patterns for goal-directed actions in chimpanzees, and to determine whether chimpanzee infants would pay attention to faces like humans [28] . Both phylogenetic and ontogenetic comparisons will provide more insights into the evolutionary origins and underlying cognition of attention allocation while viewing goal-directed actions of other individuals. Participants A total of 15 full-term 8-month-old infants (nine males, mean age=8 months and 5 days, s.d.=7 days), 14 full-term 12-month-old infants (eight males, mean age=12 months and 4 days, s.d.=8 days) and 15 adults (seven males, mean age=22.4 years, s.d.=2.3 years) participated in Experiment 1. An additional two 8-month-olds, two 12-month-olds and one human adult were tested, but excluded due to fussiness ( n =2) or inattentiveness ( n =3) during sessions. Another 13 human adults (seven males, mean age=21.5 years, s.d.=2.1 years), 15 different adults (eight males, mean age=22.5 years, s.d.=2.0 years) and 12 different adults (six males; mean age=20.9 years, s.d.=2.2 years) participated in Experiment 2, 3 and 4, respectively. The same six chimpanzees ( Pan troglodytes : two males, 5–15 years) participated in Experiment 1, 2, 3 and 4. Infants' parents and adult participants provided written consent according to guidelines specified by the Ethical Committee of the Japan Science and Technology Agency; the study was conducted in accordance with the standards specified in the 1964 Declaration of Helsinki. Care and use of chimpanzees adhered to guidelines established by the Primate Society of Japan. The study was approved by the Animal Welfare and Animal Care Committee of the Hayashibara Biochemical Laboratories, Inc. The chimpanzees were cared for at the Great Ape Research Institute, Hayashibara Biomedical Laboratories, Inc. The two males (both 15 years old) and four females (14, 14, 11 and 5 years old) lived as a group. All of them previously participated in several kinds of behavioural cognitive tasks, including tool use, sequential learning using touch screens and eye-tracking [29] . The chimpanzees spent a few hours each day interacting with humans indoors for study or husbandry purposes. They were not deprived of food for the testing. Apparatus and stimuli A Tobii (Stockholm, Sweden) T60 Eye Tracker, integrated with a 17-inch TFT monitor, was used to present stimuli and record eye movements by image processing algorithms (60 Hz; Tobii Studio 2.1. 12, Tobii Technology). Participants were seated approximately 60 cm from the monitor. Stimulus presentation and recording were controlled via a computer (Dell T7500 for humans, Dell M4400 for chimpanzees) with Tobii Studio software. The video stimuli used for experiments and AOIs for analysis are shown in Figure. 1 . The entire video subtended 21.6°×16.2° of visual angle. Before the video presentation, small animation videos were shown to the participants to direct their attention to the monitor. Procedure When the infant participants arrived at the lab, they were brought into the study room, which was softly illuminated to render the monitor screen, the most salient feature of the room. Infants were then placed on their parents' lap and were seated centrally in front of the monitor. An initial calibration procedure was conducted; this was considered successful when measures from five calibration points were obtained. This procedure was repeated until the calibration criterion was met for each infant. For human adults, the same procedure was followed, with the exception that they sat in a normal chair during the experiment. They were instructed simply to watch the video until it ended. In case of the chimpanzees, familiar human experimenters remained in the study room during testing, and one of them stood beside the chimpanzee and positioned the participant's face for the recordings while the chimpanzee sat in front of the monitor on which the eye tracker was mounted. Calibration for each chimpanzee was achieved at the beginning of the session by showing a small video clip at two calibration points. Participants were then shown a video of an actor performing an action. In Experiment 1, 2 and 4, human participants were then shown two repetitions of the video separated by an interval of approximately 4–20 s. During the interval, animations or other video clips were shown. Chimpanzee participants were shown a single video demonstration in a session, with two sessions conducted on separate days. In Experiment 3, human and chimpanzee participants were shown four repetitions of the action. The experiment relied on voluntary participation by the chimpanzees, and during testing, they showed no negative emotional expressions such as screaming or grimacing. Data analysis Fixations were scored using a Tobii fixation filter with a threshold radius of 35 pixels; statistical tests were calculated using SPSS (SPSS Inc.). We have applied parametric tests after examining the normality of our data sample by graphical inspection of a Q–Q plot for normality, and by conducting a Shapiro–Wilk test. Ratios of looking time data were analysed with angular transformation. Both latency and looking time data were averaged across the trials, resulting in one aggregated data point per participant and analysis. In Experiment 1, we defined four AOI of the same size covering, respectively: most of the trajectory of the moving bottle (Trajectory AOI), the cup (Cup AOI), the actor's face during bottle manipulation (Face AOI) and the other (control region) area (Other AOI). The goal was defined as the onset of pouring juice into the cup. Data were analysed for each of two phases, before and after goal achievement; the before-goal phase, defined from the frame at which manipulation of the bottle started to the frame showing the onset of pouring (2.6 s); and the after-goal phase, defined from the frame showing the onset of pouring until the frame showing the end of the pouring action (6.7 s). The latency of the infants' fixation shift to the Cup AOI was compared with the onset of pouring juice. If looking at the Cup AOI occurred before the onset of pouring (defined as a zero point), the trial was considered predictive. Using single-sample t -tests, latency data (in ms) were tested against the zero point to assess whether performance was significantly predictive or reactive. Latency of fixation shift to the Cup AOI was also compared across the four groups using one-way ANOVA and subsequent post-hoc tests (Bonferroni). For the analysis of the ratio of looking time to the total looking time towards the four areas combined, we conducted 2×4×4 mixed factorial ANOVAs with within-subjects factors of phase (before goal, after goal) and area (cup, face, trajectory, other), and the between-subjects factor, experimental group (8-, 12-month-olds, adults, chimpanzees), with follow-up two-way ANOVAs and subsequent post-hoc tests (Bonferroni). Number of fixations was also examined using a 4 (area)×4 (group) mixed ANOVA. Furthermore, average fixation durations were examined using a 2 (area: face, object (cup+trajectory))×4 (group) mixed ANOVA. A two-tailed Student's t -test using the Bonferroni correction was used for pairwise comparisons. For Experiment 2, we defined two AOI of the same size: one covering the moving tool (a rubber tube) and the honey container (Object AOI), and the other covering the actor's face (Face AOI). The goal was defined as the rubber tube's first contacting with the honey. Data were analysed for each of the two phases, before and after the goal was achieved: the before-goal phase, defined from the onset of the frame in which manipulation of the rubber tube began to the onset frame, showing the rubber tube making contact with the honey (4.5 s); and the after-goal phase, defined from the frame showing the rubber tube's first contact with the honey to the frame, showing the tube being withdrawn (3.0 s). Data were analysed using a 2×2×2 mixed ANOVA, with the within-subjects factors of the phase (before goal, after goal) and area (face, object), and the between-subjects factor of the group (adults, chimpanzees) for the ratio of looking time to total looking time towards the two areas combined. The number of fixations and average fixation durations were examined using a 2 (area)×2 (group) mixed ANOVA. In Experiment 3, we defined two AOIs of the same size: one covering the trajectory of hand movements plus the four objects (Object AOI) and the other covering the actor's face (Face AOI). Gaze was measured from the time the demonstrator first started to reach for an object until she withdrew her hand from the last reached object (14.1 s). To compare the ratio of looking at the face between the goal-directed action (including both phases) in Experiment 1 and the non-goal-directed action in Experiment 3, a paired t -test (two-tailed) was used for chimpanzees and an unpaired t -test (two-tailed) was used for human adults. For Experiment 4, we defined two AOI: one covering the trajectory of the moving object (Object AOI) and the other covering the actor's face (Face AOI). Gaze was measured from the time the demonstrator first started to reach for a cup until she removed her hand from the last grasped cup (the six cups were successively stacked, taking 10.6 s). The ratio of looking time towards the face area to total looking time towards the two areas combined (face+object) were compared between humans and chimpanzees using one-way ANOVA. Calibration errors In case of chimpanzees, calibration error was estimated before testing, and the average error across participants was 0.40° (s.d.=0.38°) of the visual angle of the chimpanzees [29] . We did not measure the calibration errors precisely in case of human infants and adults, because of accumulated knowledge about the validity of data collection using exactly the same device [11] , [12] , [25] , but the errors can be estimated as within the range of 1° of visual angle at most for our participants, judging from their fixation data with the stimulus used for attention getting. One degree of visual angle is larger than the difference between the outline of each feature (that is, face, cup, trajectory) and that of the respective AOI; thus, it is unlikely that calibration error affected the analysis of gaze behaviour. How to cite this article: Myowa-Yamakoshi, M. et al . Humans and chimpanzees attend differently to goal-directed actions. Nat. Commun. 3:693 doi: 10.1038/ncomms1695 (2012).